Polycomb repressive complex 2 regulates skeletal growth by suppressing Wnt and TGF-β signalling Polycomb repressive complex 2 (PRC2) controls maintenance and lineage determination of stem cells by suppressing genes that regulate cellular differentiation and tissue development. However, the role of PRC2 in lineage-committed somatic cells is mostly unknown. Here we show that Eed deficiency in chondrocytes causes severe kyphosis and a growth defect with decreased chondrocyte proliferation, accelerated hypertrophic differentiation and cell death with reduced Hif1a expression. Eed deficiency also causes induction of multiple signalling pathways in chondrocytes. Wnt signalling overactivation is responsible for the accelerated hypertrophic differentiation and kyphosis, whereas the overactivation of TGF-β signalling is responsible for the reduced proliferation and growth defect. Thus, our study demonstrates that PRC2 has an important regulatory role in lineage-committed tissue cells by suppressing overactivation of multiple signalling pathways. Most mineralized bone is formed through endochondral bone formation in which the growth plate, a cartilage template formed by chondrocytes, is continuously replaced by mineralized bone. Chondrocytes differentiate from multi-potent mesenchymal progenitors. After lineage commitment, growth plate chondrocytes go through multiple maturation steps to differentiate into post-mitotic hypertrophic chondrocytes [1] , [2] . Proliferation and differentiation of growth plate chondrocytes is tightly controlled by multiple signalling systems [3] , including Indian hedgehog, parathyroid hormone-related peptide [1] , [4] , fibroblast growth factor [2] , [5] , C-type natriuretic peptide [6] , insulin-like growth factor [7] , bone morphogenetic protein, transforming growth factor-β (TGF-β) [8] , [9] and Wnt signalling [10] , [11] . These extracellular signalling molecules are further mediated by specific and common intracellular signalling pathways, including the mitogen-activated protein kinase and phosphoinositide 3 kinase pathways. Multiple epigenetic mechanisms regulate gene expression and thus control a variety of biological processes [12] , [13] , [14] . Altering chromatin structure via histone modification is a major epigenetic mechanism affected by polycomb group proteins. Polycomb repressive complex 2 (PRC2), whose core components include Ezh1/2 (enhancer of zeste homologue1/2), Eed (embryonic ectoderm development) and Suz12 (suppressor of zeste 12 homologue), catalyses tri-methylation of lysine 27 of histone 3 (H3K27me3), and silences chromatin [15] . These three components are essential for the methyltransferase activity of PRC2. PRC2 regulates expression of the key differentiation-related genes to control differentiation of embryonic stem cells (ESCs) [14] and several tissue-specific stem/progenitor cells including haematopoietic stem cells [16] , [17] , [18] , neural stem cells [19] , [20] , muscle stem cells [21] and epidermal stem cells [22] , [23] . These findings are in line with the notion that PRC2-mediated chromatin silencing controls cell fate transition of stem/progenitor cells [24] . However, the role of PRC2 in lineage-committed somatic cells is not clear. Here we delete Eed in lineage-committed chondrocytes to investigate the role of PRC2 in skeletal development. We show that PRC2 has an essential role in regulating proliferation and differentiation of growth plate chondrocytes by suppressing multiple signalling pathways. Eed deletion in chondrocytes causes skeletal defects In order to investigate the role of PRC2 in skeletal development, we ablated the Eed gene in chondrocytes using floxed Eed mice and Col2-Cre transgenic mice in which Cre recombinase is expressed under the control of a mouse Col2a1 promoter. Eed conditional knockout ( Col2-Cre:Eedfl/fl , cKO) mice were born and survived postnatally, but showed growth impairment, shortening of long bones and severe kyphosis, and usually died by 4 weeks ( Fig. 1a–c ). The mutant thoracic spine was severely deformed ( Fig. 1d ). In addition to vertebral bodies, intervertebral discs that are also formed by cells derived from Col2a1 -positive progenitors showed a reduction in size in Eed cKO mice ( Fig. 1e ). Using primary chondrocytes isolated from ribs, we confirmed efficient elimination of Eed at the protein and RNA levels and H3K27me3 in Eed cKO chondrocytes ( Fig. 1f–h ). 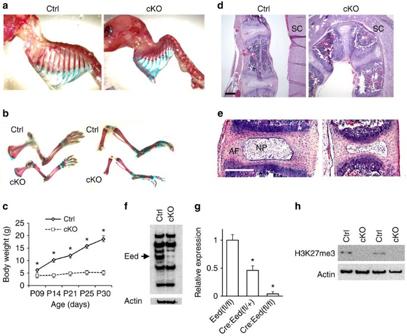Figure 1: ConditionalEeddeletion in chondrocytes causes skeletal defects. (a,b) Whole-mount skeletal preparation of littermate control (Ctrl) andEedcKO mice at P11. Both male and female cKO mice show severe kyphosis (Upper) and shortening of long bones of forelimbs (lower left) and hind limbs (lower right). (c) cKO mice show impaired growth. A majority of cKO mice dies by P21. Male and female mice were combined.n=3–6; *P<0.05 versus Ctrl, error bars show the s.e.m., unpaired Student’st-test was used. (d) Sagittal sections of thoracic vertebrae of mice at P28.5. SC, spinal cord. (e) Intervertebral discs are also affected.EedcKO mice show reduced size of the annulus fibrosus (AF) and nucleus pulposus (NP). (f) Immunoblot analysis using protein lysate of primary rib chondrocytes cultured overnight shows an efficient reduction in the Eed protein in cKO chondrocytes. The arrow indicates the signal specific to Eed. (g) TheEedRNA expression level determined by qPCR in chondrocytes from indicated genotypes. (h) H3K27me3 is absent in primary rib chondrocytes of cKO mice (Supplementary Fig. 6; the uncropped blot result images). Scale bars, 200 μm. Figure 1: Conditional Eed deletion in chondrocytes causes skeletal defects. ( a , b ) Whole-mount skeletal preparation of littermate control (Ctrl) and Eed cKO mice at P11. Both male and female cKO mice show severe kyphosis ( Upper ) and shortening of long bones of forelimbs ( lower left ) and hind limbs ( lower right ). ( c ) cKO mice show impaired growth. A majority of cKO mice dies by P21. Male and female mice were combined. n =3–6; * P <0.05 versus Ctrl, error bars show the s.e.m., unpaired Student’s t -test was used. ( d ) Sagittal sections of thoracic vertebrae of mice at P28.5. SC, spinal cord. ( e ) Intervertebral discs are also affected. Eed cKO mice show reduced size of the annulus fibrosus (AF) and nucleus pulposus (NP). ( f ) Immunoblot analysis using protein lysate of primary rib chondrocytes cultured overnight shows an efficient reduction in the Eed protein in cKO chondrocytes. The arrow indicates the signal specific to Eed. ( g ) The Eed RNA expression level determined by qPCR in chondrocytes from indicated genotypes. ( h ) H3K27me3 is absent in primary rib chondrocytes of cKO mice ( Supplementary Fig. 6 ; the uncropped blot result images). Scale bars, 200 μm. Full size image PRC2 regulates chondrocyte proliferation and differentiation While the overall structure of growth plates is relatively well preserved, Eed cKO chondrocytes of tibial growth plates and fetal vertebrae showed significant decreases in cell proliferation ( Fig. 2a–d ). This proliferation defect likely led to a reduction in the number of type X collagen ( Col10a1 )-expressing hypertrophic chondrocytes that are differentiated from proliferating chondrocytes ( Fig. 2e ). The marker of terminally differentiated hypertrophic chondrocytes, Spp1 , was found beneath the hypertrophic layer both in control and Eed cKO growth plate; however, we occasionally observed chondrocytes below the Spp1 domain, suggesting delayed cartilage resorption ( Fig. 2e ). In order to investigate the effect of Eed deficiency on chondrocyte differentiation, we examined the initial appearance of hypertrophic chondrocytes in the embryonic axial skeleton. Appearance of Col10a1 -expressing hypertrophic chondrocytes was advanced in Eed cKO mice at multiple developmental stages ( Fig. 2f ), demonstrating that Eed deficiency accelerates hypertrophic differentiation. 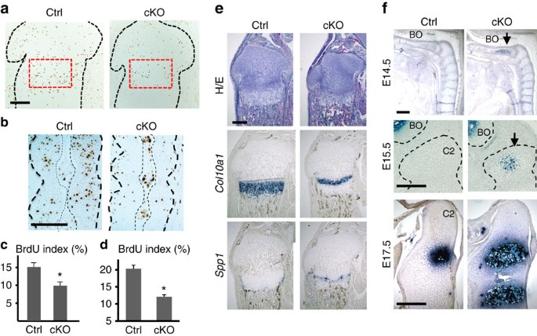Figure 2: Proliferation and differentiation defects inEed-deficient chondrocytes. (a,c) BrdU incorporation is significantly reduced in growth plate chondrocytes ofEedcKO mice. Black dotted lines indicate the contour of the proximal epiphysis of tibiae. The BrdU labelling index in the proliferating zone, indicated by red-dotted lines, was counted in P 1.5-old littermate control and cKO mice. (b,d) BrdU incorporation is significantly reduced in the cartilage anlage of the cKO spinal primordium at E15.5. Thick black dotted lines indicate the contour of the spinal primordium at the level of C4 and C5. Thin dotted lines indicate the notochord.n=3; *P<0.05 versus Ctrl. (e) TheCol10a1-expressing hypertrophic chondrocyte domain is reduced in the P1.5-old cKO tibial growth plate. An unresorbed hypertrophic chondrocyte layer beneath theSpp1domain is occasionally present in cKO mice. (f) Sagittal sections of the spine show premature differentiation ofCol10a-expressing hypertrophic chondrocytes (arrows) in cKO vertebral bones at indicated ages. BO, basi-occipital bone; C2, second cervical vertebra (axis). Scale bars, 200 μm. Figure 2: Proliferation and differentiation defects in Eed -deficient chondrocytes. ( a , c ) BrdU incorporation is significantly reduced in growth plate chondrocytes of Eed cKO mice. Black dotted lines indicate the contour of the proximal epiphysis of tibiae. The BrdU labelling index in the proliferating zone, indicated by red-dotted lines, was counted in P 1.5-old littermate control and cKO mice. ( b , d ) BrdU incorporation is significantly reduced in the cartilage anlage of the cKO spinal primordium at E15.5. Thick black dotted lines indicate the contour of the spinal primordium at the level of C4 and C5. Thin dotted lines indicate the notochord. n =3; * P <0.05 versus Ctrl. ( e ) The Col10a1 -expressing hypertrophic chondrocyte domain is reduced in the P1.5-old cKO tibial growth plate. An unresorbed hypertrophic chondrocyte layer beneath the Spp1 domain is occasionally present in cKO mice. ( f ) Sagittal sections of the spine show premature differentiation of Col10a -expressing hypertrophic chondrocytes (arrows) in cKO vertebral bones at indicated ages. BO, basi-occipital bone; C2, second cervical vertebra (axis). Scale bars, 200 μm. Full size image Eed deletion decreases Hif1a and induces cell death We also found that Eed cKO mice often showed reduced cellular density in the central area of epiphyseal growth plates at early postnatal stages ( Fig. 3a ). TdT-mediated dUTP nick end labelling staining demonstrated cell death in this region. The growth plate is a hypoxic tissue where most of the hypoxic chondrocytes are located in the centre of the columnar proliferating chondrocyte layer. The functional activity of the hypoxia-inducible transcription factor 1α (Hif1a) is required to maintain chondrocyte viability within the central region of the growth plate [25] . On the basis of the similarity in the pattern of cell death between Eed -deficient and Hif1a -deficient growth plates, we examined expression of Hif1a and the Hif1a downstream target genes. RNA expression of Hif1a and its known target genes were downregulated in Eed cKO chondrocytes at the normoxic condition ( Fig. 3b ). Protein expression levels of Hif1a and the Hif1a target, Bnip3, were decreased in cKO primary chondrocytes both in the normoxic (21% oxygen) and hypoxic (2% oxygen) conditions ( Fig. 3c ). Hypoxia-dependent Hif1a protein stabilization, a major regulatory mechanism of Hif1a expression, was intact in Eed cKO chondrocytes, since hypoxia efficiently increased the Hif1a protein level and Hif1a activity in both control and cKO chondrocytes ( Fig. 3c,e ). Thus, the reduction in Hif1a expression in Eed -deficient chondrocytes appeared to be mainly caused by a decrease in Hif1a mRNA. These findings suggest that transcriptional regulation of Hif1a by PRC2 is necessary for chondrocyte viability within the central region of the growth plate. 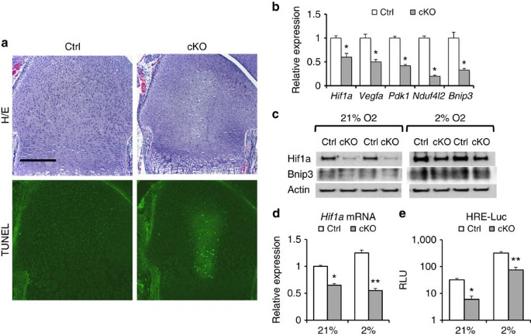Figure 3:Eeddeletion impairs hypoxic adaptation of chondrocytes. (a) Haematoxylin/eosin (top) and TdT-mediated dUTP nick end labeling (TUNEL;bottom)-stained sections of the distal femoral growth pate of P1.5-old mice. Cell death is detected in the central area of theEedcKO growth plate. (b) Expression levels ofHif1aand indicated Hif1a target genes were reduced in primaryEedcKO chondrocytes cultured in the normoxic condition. RNA expression levels were determined by qRT–PCR. Expression levels were normalized toActblevels.n=4; *P<0.05 versus Ctrl. (c) Expression of Hif1a and Bnip3 is reduced in primary cKO rib chondrocytes both in normoxic (21% O2) and hypoxic (2% O2) conditions. (d) TheHif1amRNA level is significantly reduced in cKO chondrocytes.Hif1alevels were normalized by 18S ribosomal RNA.n=4; *P<0.05, **P<0.01 versus Ctrl. (e) Hif1a activity, assessed by a Hif1a-responsive luciferase reporter (HRE-luc), was reduced in cKO in both normoxic and hypoxic conditions.n=6; *P<0.05, **P<0.01 versus Ctrl. Scale bars, 200 μm. Error bars show the s.e.m., unpaired Student’st-test was used. Figure 3: Eed deletion impairs hypoxic adaptation of chondrocytes. ( a ) Haematoxylin/eosin ( top ) and TdT-mediated dUTP nick end labeling (TUNEL; bottom )-stained sections of the distal femoral growth pate of P1.5-old mice. Cell death is detected in the central area of the Eed cKO growth plate. ( b ) Expression levels of Hif1a and indicated Hif1a target genes were reduced in primary Eed cKO chondrocytes cultured in the normoxic condition. RNA expression levels were determined by qRT–PCR. Expression levels were normalized to Actb levels. n =4; * P <0.05 versus Ctrl. ( c ) Expression of Hif1a and Bnip3 is reduced in primary cKO rib chondrocytes both in normoxic (21% O 2 ) and hypoxic (2% O 2 ) conditions. ( d ) The Hif1a mRNA level is significantly reduced in cKO chondrocytes. Hif1a levels were normalized by 18S ribosomal RNA. n =4; * P <0.05, ** P <0.01 versus Ctrl. ( e ) Hif1a activity, assessed by a Hif1a-responsive luciferase reporter (HRE-luc), was reduced in cKO in both normoxic and hypoxic conditions. n =6; * P <0.05, ** P <0.01 versus Ctrl. Scale bars, 200 μm. Error bars show the s.e.m., unpaired Student’s t -test was used. Full size image PRC2 controls activities of multiple signalling pathways To understand the molecular mechanism, first we performed chromatin immunoprecipitation (ChIP) followed by sequencing (ChIP-seq) to identify genes that carried the H3K27me3 mark in chondrocytes (Gene Expression Omnibus (GEO) #GSE67132 and #GSE76467; Supplementary Data 1 ). We found that 3,925 genes were associated with H3K27me3 in chondrocytes ( Supplementary Fig.1a and Supplementary Data 1 ). As found in ESCs [26] , genes encoding transcription factors and signalling molecules were preferred PRC2 targets in chondrocytes as well. We also performed gene expression analysis to identify genes whose expression was altered upon Eed deletion (GEO #GSE66862). We found that 1,817 annotated genes were upregulated more than 1.25-fold in Eed -null chondrocytes ( Supplementary Fig. 1 and Supplementary Data 2 ). Among these, 433 genes carried the H3K27me3 mark, suggesting that the majority of deregulated genes in Eed -deficient chondrocytes were indirectly regulated by PRC2 ( Supplementary Data 1 ). The finding that only 433 among 3,925 genes marked with H3K27me3 were derepressed in Eed -deficient chondrocytes also suggests that a majority of PRC2 target genes are repressed by other mechanisms. Since genes encoding signalling molecules account for a considerable fraction of H3K27me3-marked genes in chondrocytes, we determined the basal signalling status of major signalling pathways in Eed -deficient chondrocytes. We found that Eed deficiency caused overactivation in multiple signalling pathways ( Fig. 4a–c and Supplementary Fig. 2b ). Phosphorylation of signalling molecules of the extracellular-signal-regulated kinase (ERK), p38 mitogen-activated protein kinase, phosphoinositide 3 kinase and TGF-β pathways was upregulated. Increases in active β-catenin and Wnt reporter activity indicated the upregulation of canonical Wnt signalling in Eed -deficient chondrocytes ( Fig. 4a,b,g ). We also found a modest upregulation in retinoic acid (RA) signalling assessed by a luciferase reporter assay. As found in the microarray analysis ( Supplementary Data 2 ), we found upregulation in Wnt10a and Lef1 , of which genomic loci were associated with H3K27me3 ( Fig. 4e and Supplementary Fig. 1b ), and the Wnt target gene, Axin2 ( Fig. 4d ). We also found upregulation of Wnt receptors, including Fzd6 and Lrp5 ( Fig. 4d ); however, these genes did not carry the H3K27me3 mark, suggesting that PRC2 loss indirectly increased expression of these genes. With regard to the TGF-β signalling pathway, we found that Tgfbr2 was upregulated at both mRNA and protein levels ( Fig. 4a,d,f ). We did not find significant H3K27me3 modification at the Tgfbr2 gene locus; thus, Tgfbr2 upregulation in chondrocytes is likely an indirect consequence of the loss of PRC2 function. 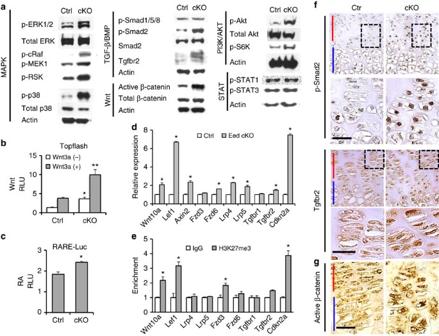Figure 4:Eeddeletion causes aberrant activation of multiple signalling pathways. (a) The basal levels of major signalling pathways in primary rib chondrocytes were determined by immunoblot analysis using indicated phospho-specific antibodies. (b) Topflash Wnt reporter assay shows upregulation of Wnt activity in cKO chondrocytes both at the basal and Wnt3a-stimulated conditions. After transfection, cells were cultured with or without Wnt3a (20 ng ml−1) for 24 h.n=6; *P<0.05, **P<0.01 versus Ctrl. (c) RA-responsive luciferase assay (RARE-Luc) shows modest upregulation in RA signalling in cKO chondrocytes.n=6; *P<0.05 versus Ctrl. (d) RNA expression of indicated genes in primary rib chondrocytes were determined by qRT–PCR.n=4; *P<0.05 versus Ctrl. (e) H3K27me3 ChIP-PCR analysis of indicated genes.n=4; *P, 0.05 versus IgG control. (f) Immunostaining for p-Smad2 and Tgfbr2 on tibial growth plate sections of Ctrl and cKO mice. Representative pictures of three independent experiments are shown. (g) Immunostaining for non-phosphorylated β-catenin (active form) on tibial growth plate sections from Ctrl and cKO. Representative pictures of three independent experiments are shown. Red bar indicates the proliferating chondrocyte zone and blue bar indicates the hypertrophic chondrocyte zone of the growth plate. Scale bars, 20 μm. Error bars show the s.e.m., unpaired Student’st-test was used. Figure 4: Eed deletion causes aberrant activation of multiple signalling pathways. ( a ) The basal levels of major signalling pathways in primary rib chondrocytes were determined by immunoblot analysis using indicated phospho-specific antibodies. ( b ) Topflash Wnt reporter assay shows upregulation of Wnt activity in cKO chondrocytes both at the basal and Wnt3a-stimulated conditions. After transfection, cells were cultured with or without Wnt3a (20 ng ml −1 ) for 24 h. n =6; * P <0.05, ** P <0.01 versus Ctrl. ( c ) RA-responsive luciferase assay (RARE-Luc) shows modest upregulation in RA signalling in cKO chondrocytes. n =6; * P <0.05 versus Ctrl. ( d ) RNA expression of indicated genes in primary rib chondrocytes were determined by qRT–PCR. n =4; * P <0.05 versus Ctrl. ( e ) H3K27me3 ChIP-PCR analysis of indicated genes. n =4; * P , 0.05 versus IgG control. ( f ) Immunostaining for p-Smad2 and Tgfbr2 on tibial growth plate sections of Ctrl and cKO mice. Representative pictures of three independent experiments are shown. ( g ) Immunostaining for non-phosphorylated β-catenin (active form) on tibial growth plate sections from Ctrl and cKO. Representative pictures of three independent experiments are shown. Red bar indicates the proliferating chondrocyte zone and blue bar indicates the hypertrophic chondrocyte zone of the growth plate. Scale bars, 20 μm. Error bars show the s.e.m., unpaired Student’s t -test was used. Full size image TGF-β suppression rescues proliferation and growth defects Because the ERK, p38 and TGF-β pathways, which were upregulated in Eed cKO chondrocytes, were shown to regulate endochondral bone growth [27] , [28] , [29] , [30] , we inhibited these signalling pathways in vivo to test whether upregulation of these signalling pathways contributed to the skeletal abnormalities of Eed cKO mice. Whereas inhibition of the ERK or p38 signalling pathway had no effects on the skeletal defects of Eed cKO mice ( Supplementary Fig. 2c ), inhibition of TGF-β signalling using the TGF-β receptor inhibitor, Ly364947, ameliorated the growth defect during early postnatal stages ( Fig. 5a ). Analysis of the growth plate of Eed cKO mice treated with Ly364947 revealed a decrease in phospho-Smad2 immunostaining and a significant increase in chondrocyte proliferation compared with vehicle-treated Eed cKO mice ( Fig. 5b and Supplementary Fig. 4d ). We also assessed the effect of TGF-β signalling suppression on chondrocyte proliferation in vitro . TGF-β signalling inhibition using TGF-β receptor inhibitor (Ly364947) or neutralizing antibody against TGF-β ligands (1D11) significantly ameliorated proliferation defect of Eed cKO chondrocytes in vitro ( Fig. 5c,d ). Because Tgfbr2 was significantly upregulated in Eed cKO chondrocytes, to test whether upregulation of Tgfbr2 was responsible for the proliferation defect of Eed cKO chondrocytes, we knocked down Tgfbr2 using retroviruses expressing small hairpin RNAs (shRNAs) in primary rib chondrocytes in vitro . With ∼ 60% infection efficiency, Tgfbr2 expression was reduced by 40–60% ( Supplementary Fig. 5a ). Tgfbr2 knockdown in Eed cKO chondrocytes showed a significant increase in proliferation in vitro ( Fig. 5e,f ). We also found that the well-known PRC2 target, Cdkn2a ( Ink4a/Arf ), encoding negative cell cycle regulators [31] was upregulated in Eed cKO chondrocytes ( Fig. 4d,e ). To evaluate the role of Cdkn2a upregulation in chondrocyte proliferation, we knocked down Cdkn2a in Eed cKO chondrocytes; Cdkn2a knockdown had little effect in chondrocytes unlike Tgfbr2 knockdown despite the similar knockdown efficiencies ( Supplementary Fig. 5b,c ). 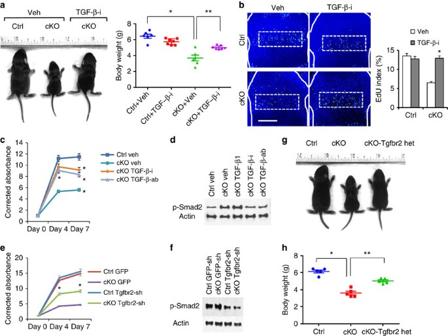Figure 5: TGF-β inhibition rescues the growth defect ofEedcKO mice. (a) The TGF-β receptor inhibitor, Ly364947, was injected daily into pregnant or nursing mothers from E14.5 through P7.5. Mice at P7.5 are shown. Body weight was measured at P7.5.n≥6; *P<0.05 versus Ctrl, **P<0.05 versus vehicle-treated cKO. (b) EdU staining of proximal tibial growth plates. The fraction of EdU-positive nuclei was calculated in proliferating columnar chondrocyte zone (dotted lines). White solid lines indicate the epiphyseal bone contour.n=3; *P<0.05 versus vehicle-treated cKO mice. Scale bars, 200 μm. (c) Cell proliferation assay on primary chondrocytes isolated from wild-type (Ctrl) andEedcKO (cKO) mice, treated with dimethylsulphoxide (DMSO; Veh) or a TGF-β receptor inhibitor (TGF-β-i; Ly364947, 0.2 μM), TGF-β ligand-neutralizing antibody (TGF-β-ab; 5 μg ml−1) or TGF-β1 (20 ng ml−1). Treatment with Ly364947 and TGF-β-ab significantly ameliorated the proliferation defect of cKO cells.n=3; *P<0.01 and **P<0.05. (d) Treatment with TGF-β-i and TGF-β-ab decreases the p-Smad2 level. (e) Primary rib chondrocytes from Ctrl and cKO mice were infected with retroviruses expressingTgfbr2shRNA (Tgfbr2-sh) or eGFP (enhanced green fluorescent protein; GFP). Tgfbr2 knockdown using Tgfbr2-sh2 virus in cKO chondrocytes significantly increases proliferation.n=6; *P<0.05. (f) The p-Smad level is decreased inTgfbr2knockdown chondrocytes. (g)Tgfbr2heterozygosity (cKO-Tgfbr2het) significantly improves animal growth ofEedcKO mice. (h) Body weight of control (Ctrl),EedcKO (cKO) andEedcKO mice missing one allele ofTgfbr2(cKO-Tgfbr2het) was measured at P7.5. Mice with conditionalTgfbr2heterozygous deletion alone (Col2-Cre:TgfbrloxP/+) show no noticeable skeletal abnormalities, as also previously described37.n≥5; *P<0.01 and **P<0.05. Error bars show the s.e.m., unpaired Student’st-test was used. Figure 5: TGF-β inhibition rescues the growth defect of Eed cKO mice. ( a ) The TGF-β receptor inhibitor, Ly364947, was injected daily into pregnant or nursing mothers from E14.5 through P7.5. Mice at P7.5 are shown. Body weight was measured at P7.5. n≥ 6; * P <0.05 versus Ctrl, ** P <0.05 versus vehicle-treated cKO. ( b ) EdU staining of proximal tibial growth plates. The fraction of EdU-positive nuclei was calculated in proliferating columnar chondrocyte zone (dotted lines). White solid lines indicate the epiphyseal bone contour. n =3; * P <0.05 versus vehicle-treated cKO mice. Scale bars, 200 μm. ( c ) Cell proliferation assay on primary chondrocytes isolated from wild-type (Ctrl) and Eed cKO (cKO) mice, treated with dimethylsulphoxide (DMSO; Veh) or a TGF-β receptor inhibitor (TGF-β-i; Ly364947, 0.2 μM), TGF-β ligand-neutralizing antibody (TGF-β-ab; 5 μg ml −1 ) or TGF-β1 (20 ng ml −1 ). Treatment with Ly364947 and TGF-β-ab significantly ameliorated the proliferation defect of cKO cells. n =3; * P <0.01 and ** P <0.05. ( d ) Treatment with TGF-β-i and TGF-β-ab decreases the p-Smad2 level. ( e ) Primary rib chondrocytes from Ctrl and cKO mice were infected with retroviruses expressing Tgfbr2 shRNA ( Tgfbr2 -sh) or eGFP (enhanced green fluorescent protein; GFP). Tgfbr2 knockdown using Tgfbr2-sh2 virus in cKO chondrocytes significantly increases proliferation. n =6; * P <0.05. ( f ) The p-Smad level is decreased in Tgfbr2 knockdown chondrocytes. ( g ) Tgfbr2 heterozygosity (cKO- Tgfbr2 het) significantly improves animal growth of Eed cKO mice. ( h ) Body weight of control (Ctrl), Eed cKO (cKO) and Eed cKO mice missing one allele of Tgfbr2 (cKO- Tgfbr2 het) was measured at P7.5. Mice with conditional Tgfbr2 heterozygous deletion alone ( Col2 - Cre:Tgfbr loxP/+ ) show no noticeable skeletal abnormalities, as also previously described [37] . n ≥5; * P <0.01 and ** P <0.05. Error bars show the s.e.m., unpaired Student’s t -test was used. Full size image To further investigate the role of the Tgfbr2 upregulation in Eed cKO mice in vivo , we generated compound conditional mutant mice missing Eed and one allele of Tgfbr2 . Tgfbr2 heterozygosity significantly improved cellular proliferation and animal growth in Eed cKO mice ( Fig. 5g,h and Supplementary Fig. 5d ). These results demonstrate that the overactivation of TGF-β signalling because of the upregulation of Tgfbr2 plays a causal role for the proliferation defect of growth plate chondrocytes and growth impairment of Eed cKO mice. Wnt signalling overactivation causes kyphosis Although TGF-β inhibition rescued the growth defect, inhibition of the TGF-β, ERK or p38 signalling pathways did not improve the spinal deformity ( Supplementary Fig. 2c ). Because the Wnt pathway, which was also upregulated in Eed cKO chondrocytes, was shown to regulate cartilage development by controlling chondrocyte differentiation [11] , [29] , [30] , we inhibited Wnt signalling using the porcupine inhibitor, C59. Daily treatment of C59 during fetal and neonatal stages significantly ameliorated the spinal deformity ( Fig. 6a,b ). Analysis of developing vertebrae of Eed cKO mice treated with C59 revealed significant suppression of premature hypertrophic differentiation in cKO mice ( Fig. 6e ). C59 treatment also rescued the premature closure of the growth plate between the vertebral body and transverse processes in the Eed cKO spine ( Supplementary Fig. 3a ). We confirmed that C59 treatment efficiently suppressed canonical Wnt signalling in Eed -deficient chondrocytes in vivo and in vitro ( Fig. 6c,d ). In long bones, although Wnt inhibitor treatment rescued premature hypertrophic differentiation in the secondary ossification centre of the Eed -deficient tibial epiphysis ( Supplementary Fig. 3b ), it did not rescue the growth defect ( Supplementary Fig. 3c ) or the cell proliferation defect ( Supplementary Fig. 3d ). 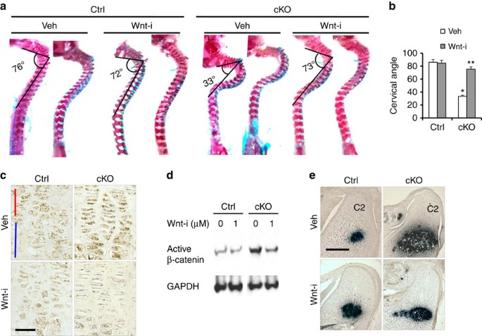Figure 6: Wnt inhibition rescues kyphosis ofEedcKO mice. (a) The effect of Wnt inhibition on kyphosis was assessed by the spinal cervical angle in P7.5-old mice. C59 Wnt inhibitor (Wnt-i) treatment from E14.5 through P7.5 significantly ameliorated kyphosis inEedcKO mice. (b) Cervical angle measurements. *P<0.05 versus vehicle-treated Ctrl. **P<0.05 versus vehicle-treated cKO. Error bars show the s.e.m., unpaired Student’st-test was used. (c) Expression of active (non-phosphorylated) β-catenin of growth plate sections of Ctrl and cKO mice was assessed 6 h after C59 (Wnt-i) or vehicle injection. A significant reduction of active β-catenin protein was observed in C59-treated animals. Scale bar, 20 μm; red bar indicates the proliferating chondrocyte zone and blue bar indicates the hypertrophic zone. (d)In vitrotreatment with C59 (Wnt-i) decreased the active (non-phosphorylated) β-catenin level inEedcKO primary rib chondrocytes. Chondrocytes were cultured for 24 h in the presence of C59 (Wnt-i). (e)Col10a1 in situhybridization on sagittal sections of the cervical spine of E17.5 embryos shows suppression of accelerated hypertrophic differentiation. C59 was injected into pregnant mothers from E 14.5 through E 17.5. C2, second cervical vertebra. Scale bar, 200 μm. Figure 6: Wnt inhibition rescues kyphosis of Eed cKO mice. ( a ) The effect of Wnt inhibition on kyphosis was assessed by the spinal cervical angle in P7.5-old mice. C59 Wnt inhibitor (Wnt-i) treatment from E14.5 through P7.5 significantly ameliorated kyphosis in Eed cKO mice. ( b ) Cervical angle measurements. * P <0.05 versus vehicle-treated Ctrl. ** P <0.05 versus vehicle-treated cKO. Error bars show the s.e.m., unpaired Student’s t -test was used. ( c ) Expression of active (non-phosphorylated) β-catenin of growth plate sections of Ctrl and cKO mice was assessed 6 h after C59 (Wnt-i) or vehicle injection. A significant reduction of active β-catenin protein was observed in C59-treated animals. Scale bar, 20 μm; red bar indicates the proliferating chondrocyte zone and blue bar indicates the hypertrophic zone. ( d ) In vitro treatment with C59 (Wnt-i) decreased the active (non-phosphorylated) β-catenin level in Eed cKO primary rib chondrocytes. Chondrocytes were cultured for 24 h in the presence of C59 (Wnt-i). ( e ) Col10a1 in situ hybridization on sagittal sections of the cervical spine of E17.5 embryos shows suppression of accelerated hypertrophic differentiation. C59 was injected into pregnant mothers from E 14.5 through E 17.5. C2, second cervical vertebra. Scale bar, 200 μm. Full size image The genome-wide mapping of PRC2-binding sites and H3K27 tri-methylation in ESCs revealed that PRC2 regulate numerous genes encoding the key developmental regulators, demonstrating the critical role of PRC2 in developmental and cellular differentiation processes [32] , [33] , [34] . While the role of PRC2 in embryonic and tissue-specific stem/progenitor cells has been extensively studied [14] , its role in lineage-committed, differentiated somatic cells is largely unexplored. The role of PRC2 in mesenchymal stem/progenitor cells of the skeletal system has been investigated in multiple models. Ezh2 deficiency in the early limb mesenchymal stem/progenitor cells reduces their proliferation, increases cell death and alters anteroposterior specification presumably because of the deregulation of patterning-regulating genes, such as Hox genes [35] . Likewise, Ezh2 deletion in neural crest cells causes derepression of Hox genes, impairs differentiation of osteochondro progenitors and results in craniofacial defects [36] . However, specific roles of PRC2 in lineage-committed, skeletal cells are not demonstrated by these studies. In this study we show that PRC2 continuously plays an important role in regulation of cellular function of chondrocytes after lineage commitment by suppressing multiple signalling pathways. Major skeletal phenotypes of Eed cKO mice include a growth defect and kyphosis. The observation that Wnt inhibitor treatment significantly ameliorated the accelerated chondrocyte differentiation and spinal deformity of Eed cKO mice strongly suggests that premature differentiation into post-mitotic hypertrophic differentiation plays a causal role for kyphosis. The acceleration of hypertrophic differentiation likely reduces the net number of chondrocytes, induces premature ossification and thus compromises spinal development. In contrast to Wnt inhibition, while TGF-β inhibitor treatment did not rescue the spinal deformity, it did rescue the proliferation defect and the growth defect in Eed cKO mice; thus, suppression of TGF-β signalling by PRC2 is essential for normal chondrocyte proliferation and animal growth. This finding is in line with previous studies in which TGF-β treatment decreases and its inhibition increases chondrocyte proliferation in vivo [27] , [28] . It is worth pointing out that the effect of TGF-β signalling on chondrocyte proliferation is likely bitropic, as Tgfbr2 conditional deletion can also reduce chondrocyte proliferation possibly depending on the differentiation status [37] , [38] . We also found that treatment of the TGF-β inhibitor at higher concentrations decreased chondrocyte proliferation as opposed to lower doses, suggesting a dose-dependent effect of TGF-β signalling on chondrocyte proliferation ( Supplementary Fig. 5e ). PRC2 is known to regulate cell proliferation by suppressing cell cycle inhibitors, such as Cdkn2a ( Ink4a/ Arf), and [16] , [18] Cdkn2a deletion partially rescues phenotypes caused by PRC2 deficiency [16] , [18] . We indeed found that Cdkn2a was upregulated in Eed cKO chondrocytes. Although we were not able to rescue the proliferation defect of Eed cKO chondrocytes by shRNA-mediated Cdkn2a knockdown in vitro , it is still possible that upregulation of cell cycle inhibitors contributes to the proliferation defect of Eed cKO chondrocytes in vivo . Nevertheless, our data demonstrate the central role of the TGF-β upregulation in the proliferation defect of Eed cKO chondrocytes. Another unique phenotype of chondrocyte-specific Eed cKO mice is the cell death in the central region of the growth plate. The central region of the growth plate is hypoxic, and hypoxia adaptation via Hif1a is essential for chondrocyte survival in this area [25] . The Hif1a level is mainly controlled at the post-transcriptional level by oxygen-dependent protein [39] . Relatively little is known about transcriptional regulation of Hif1a expression except that a few signalling pathways, such as RA [40] , NF-κB [41] and calcineurin/NFATc pathways [42] , were reported to regulate Hif1a transcription. We tested the effects of pathway-specific inhibitors on Hif1a expression in control and Eed cKO primary chondrocytes ( Supplementary Fig. 4a ). We were not able to restore expression of Hif1a or Hif1a target genes by inhibiting signalling pathways that were upregulated in Eed -deficient chondrocytes. Thus, the mechanism by which Eed deficiency decreases Hif1a transcripts is not clear at the moment. An association between chondrocyte death and TGF-β signalling was also reported in mice missing Smad7, a negative regulator of TGF-β and bone morphogenetic protein signaling, in growth plates [43] . However, Smad7 deficiency showed an increase in Hif1a protein expression, and therefore the cell death in the Smad7-null growth plate is likely caused by the Hif1a-independent mechanism. We found that TGF-β inhibition in vivo decreased the occurrence of cell death in Eed cKO mice ( Supplementary Fig. 5 ); thus, it is possible that cell death in the Eed cKO growth plate is caused by a Hif1a-independent, TGF-β signalling-dependent pathway. We demonstrate that upregulation of Tgfbr2 expression is, at least in part, responsible for growth and proliferation defects of Eed cKO mice. This finding is in line with a recent study showing that PRC2 targets and suppresses Tgfbr2 to facilitate mesenchymal–epithelial transition during reprogramming of fibroblasts into pluripotent stem cells [44] . However, we found that the Tgfbr2 gene was not strongly marked with H3K27me3 ( Supplementary Data 1 ); thus, its upregulation is likely indirectly caused by Eed deficiency in chondrocytes. Wnt signalling plays an important role during endochondral development. Ablation of β-catenin (Ctnnb1), a critical mediator of the canonical Wnt signalling pathway, in growth plate chondrocytes delays hypertrophic differentiation [45] , whereas overexpression of a stable form of Ctnnb1 in chondrocytes accelerates it [11] . In this study, we found that inhibition of Wnt signalling rescued the acceleration of hypertrophic differentiation and kyphosis in Eed cKO mice, demonstrating the critical role of PRC2-mediated suppression of Wnt signalling in regulation of chondrocyte differentiation and normal skeletal development. In summary, this work demonstrates that the PRC2 continuously plays an important regulatory role in differentiation and proliferation of lineage-committed growth plate chondrocytes by suppressing Wnt and TGF-β signalling pathways ( Fig. 7 ). 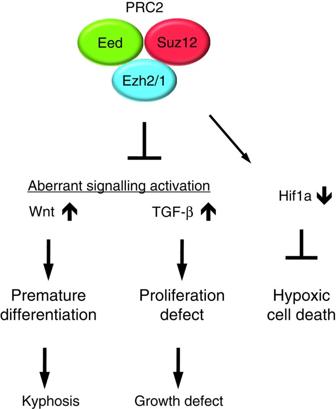Figure 7: Signalling regulation by PRC2 in chondrocytes. PRC2 is necessary for normal skeletal growth. Derepression of PRC2 target genes causes aberrant overactivation of multiple signalling systems and reducesHif1aexpression. Overactivation of Wnt and TGF-β signalling pathways is primarily responsible for the skeletal abnormalities of mice withEed-deficient chondrocytes. Figure 7: Signalling regulation by PRC2 in chondrocytes. PRC2 is necessary for normal skeletal growth. Derepression of PRC2 target genes causes aberrant overactivation of multiple signalling systems and reduces Hif1a expression. Overactivation of Wnt and TGF-β signalling pathways is primarily responsible for the skeletal abnormalities of mice with Eed -deficient chondrocytes. Full size image Mice Col2-Cre transgenic mice [46] , floxed Eed mice [18] and floxed Tgfbr2 mice [47] were previously described. Mice were in a mixed genetic background. Comparison between control and cKO mice was always made between littermates. The MEK1 inhibitor, U0126, the p38 inhibitor, SB203580, the TGF-β receptor inhibitor, LY364947, and the Wnt inhibitors, C59 and XAV-939, were purchased from Selleckchem. The RA inhibitors, BMS493 and AGN193109, were purchased from Santa Cruz Biotechnology Inc. The neutralizing antibody against TGF-β ligands, 1D11, was purchased from R&D Systems. Inhibitors were first dissolved in dimethylsulphoxide according to the manufacturer’s instructions, then diluted into 100 μl PBS and then injected daily into pregnant as well as nursing mothers intraperitoneally from E 14.5 through P9.5. The animal experiments were approved by the Institutional Animal Care and Use Committee of the Massachusetts General Hospital and performed in accordance with the regulations and guidelines. Skeletal preparation and histological analysis Skeletal preparation [48] , histological staining of paraffin-processed samples [49] and in situ hybridization [50] were performed using standard procedures. Kyphosis was assessed as previously described [51] ; two lines were drawn from the vertebral body of the first thoracic vertebra (Th1) to the spinous process of the second cervical vertebra (C2) and that of Th12; the angle formed by these two lines were measured. Proliferation and cell death assays For bromodeoxyuridine (BrdU) or ethynyldeoxyuridine (EdU) labelling, 50 μg g −1 body weight of BrdU or 20 μg g −1 of EdU was injected into mice intraperitoneally 2 h before killing. BrdU or EdU was detected using the BrdU In Situ Staining Kit or Click-iT EdU Alexa Fluor 488 Imaging Kit (Life Technologies). The BrdU or EdU labelling index was calculated as the ratio of BrdU- or EdU-positive nuclei over total nuclei in columnar proliferating chondrocytes of the growth plate. Cell death was evaluated on sections using the In Situ Cell Death Detection Kit (Roche) according to the manufacturer’s instruction. In vitro cell proliferation assay was performed using the PrestoBlue cell viability reagent (Invitrogen). Primary chondrocyte isolation and culture Primary rib chondrocytes were isolated from neonatal mice by collagenase digestion as previously described [52] . After overnight culture in DMEM containing 10% fetal calf serum, cells were subjected to downstream analysis. Luciferase reporter assay For luciferase assay, cells were trypsinized, replated in 96-well culture dishes and transfected with the 0.2 μg of Hif1a reporter (HRE-luc) [53] , the Topflash Wnt reporter [54] or a RA signalling reporter plasmid (RARE-luc) [55] and 0.02 μg of a renilla control vector using the Attractene Transfection Reagent (Qiagen). Luciferase and renilla activities were measured 48 h after transfection using the Dual-Luciferase Reporter Assay System (Promega). Quantitative reverse transcription polymerase chain reaction (qRT–PCR) RNA was extracted from primary rib chondrocytes that isolated from neonatal mice using the Direct-zol RNA Mini-Prep Kit (Zymo Research). Quantitative reverse transcription polymerase chain reaction (qRT–PCR), RNA was reverse-transcribed using DyNAmo cDNA Synthesis Kit (Life Technologies) and real-time PCR was performed using the StepOnePlus Real-time PCR system (Life Technologies) and FirePol EvaGreen qPCR mix (Solis Biodyne). Values were normalized by Actb. Primer sequences of qRT–PCR primers are as follows: Actb, 5′-GCACTGTGTTGGCATAGAGG-3′ and 5′-GTTCCGATGCCCTGAGGCTCTT-3′; 18S ribosomal RNA, 5′-AAACGGCTACCACATCCAAG-3′ and 5′-CCTCCAATGGATCCTCGTTA-3′; Hif1a, 5′-TCAAGTCAGCAACGTGGAAG-3′ and 5′-TATCGAGGCTGTGTCGACTG-3′; Vegfa, 5′-GAGAGAGGCCGAAGTCCTTT-3′ and 5′-TTGGAACCGGCATCTTTATC-3′; Pdk1, 5′-GAAGCAGTTCCTGGACTTCG-3′ and 5′-CCAACTTTGCACCAGCTGTA-3′; Ndufa4l2, 5′-TGATTGGCTTCATCTGCTTG-3′ and 5′-ACTGGTCATTGGGACTCAGG-3′; Bnip3, 5′-GGGTTTTCCCCAAAGGAATA-3′ and 5′-GAATCCTCATCCTGCAAAGC-3′; Axin2, 5′-CTCCCCACCTTGAATGAAGA-3′ and 5′-ACTGGGTCGCTTCTCTTGAA-3′; Lef1, 5′-TCACTGTCAGGCGACACTTC-3′ and 5′-TGAGGCTTCACGTGCATTAG-3′; Tgfb1r, 5′-ACCTTCTGATCCATCGGTTG-3′ and 5′-CCTGTTGGCTGAGTTGTGAC; Tgfbr2, 5′-TCGGATGTGGAAATGGAAG-3′ and 5′-CTGGCCATGACATCACTGTT-3′; Wnt10a, 5′-CCACTCCTGGCCTGTCAC-3′ and 5′-AGCCAGCAGCAGTAGGAAGA-3′; Frz3, 5′-GGTGTCCCGTGGCCTGAAG-3′ and 5′-ACGTGCAGAAAGGAATAGCCAAG-3′; Frz6, 5′-CTTTTTGATGCGGAAAGGAG-3′ and 5′-TCTTACGAGGGGCAGAAGAA-3′; Lrp4, 5′-GAATGTGCTGAGGAGGGGTA-3′ and 5′-TTGGCAAACAGTAGCACAGG-3′; Lrp5, 5′-CTGTGGCTGTGCTTCACACT-3′ and 5′-CTTGTCCAGCGGGTCATAGT-3′; Cdkn2a 5′-GTACCCCGATTCAGGTGATG-3′ and 5′-GGAGAAGGTAGTGGGGTCCT-3′. Chromatin immunoprecipitation ChIP was performed using the SimpleChIP Enzymatic Chromatin IP kit (#9003, Cell Signaling Technology), anti-H3K27me3 antibody (#9733, Cell Signaling Technology) and IgG. ChIP-ed DNA was quantified with qPCR. PCR primers used for qPCR are as follows: Wnt10a, 5′-CCACTCCTGGCCTGTCAC-3′ and 5′-AGCCAGCAGCAGTAGGAAGA-3′; Lef1, 5′-GCGAAAGGGAAGGAAAGAAG-3′ and 5′-GGATGCTGATTTCGGTGATT-3′; Lrp4, 5′-GAATGTGCTGAGGAGGGGTA-3′ and 5′-TTGGCAAACAGTAGCACAGG-3′; Lrp5, 5′-GCCGGACGACATGGAAAC-3′ and 5′-GGGACCAAGCTGCAGTACA-3′; Fzd3, 5′-CGGACTTTGCAAGAAGGACT-3′ and 5′-CCTGGCGTCCTAGGTGATAG-3′; Fzd6, 5′-GCCAGACTCCCCGAGTTAAT-3′ and 5′-ACACTTTCCGTTCTGGAAGC-3′; Tgfbr1, 5′-CCCCTCGAGCAGTTACAAAG-3′ and 5′-CCACCAACACGATGAGGAG-3′; Tgfbr2, 5′-CCGGGTAAAGTTGATGAGTGA-3′ and 5′-CCTTTACTCCTCGCCCTCTC-3′; Cdkn2a, 5′-ATCTGGAGCAGCATGGAGTC-3′ and 5′-GGGGTACGACCGAAAGAGTT-3′. More information is available in the Supplementary Methods . Western blot analysis Anti-Eed antibody (#09-774, rabbit polyclonal, 1:1,000) was purchased from Millipore. Anti-H3K27me3 antibody (GTX1121184, rabbit polyclonal, 1:500) was purchased from GeneTex. Anti-Actin antibody (I-19, rabbit polyclonal, 1:500) was purchased from Santa Cruz Biotechnology. Anti-Hif1a antibody (NB100-449, rabbit polyclonal, 1:500) was purchased from Novus Biologicals. Anti-Bnip3 antibody (ab10433, mouse monoclonal (ANa40), 2 μg ml −1 ) was purchased from Abcam. Anti-p-ERK1/2 antibody (#4370, rabbit monoclonal, 1:1,000), anti-p-MEK1 antibody (#9154, rabbit monoclonal, 1:1,000), anti-p-cRaf antibody (#9427, rabbit monoclonal, 1:1,000), anti-p-RSK antibody (#9335, rabbit monoclonal, 1:1,000) and anti-p-p38 antibody (#4511, rabbit monoclonal, 1:1,000), anti-total ERK antibody (#9102, rabbit polyclonal, 1:1,000), anti-p-Smad1/5/8antibody (#9511, rabbit polyclonal; 1:1,000), anti-Smad2 antibody (#5339, rabbit monoclonal, 1:1,000), anti-p-Smad2 antibody (#3104, rabbit polyclonal, 1:1,000), anti-TGF-β receptor II antibody (#3713, rabbit polyclonal, 1:1,000), anti-p-STAT1 antibody (#9171, rabbit polyclonal, 1:1,000) and anti-pSTAT3 antibody (#9145, rabbit monoclonal, 1:2,000) were purchased from Cell Signaling Technology. Western blot analysis was performed according to the standard procedure. Immunohistochemistry Immunohistochemistry was performed on paraffin sections using Perkin Elmer Tyramide Signal Amplification Kit (# NEL700A001KT) according to the manufacturer’s instruction. Anti-p-Smad2 (#3104, rabbit polyclonal, 1:200), anti-Tgfbr2 (#3713, rabbit polyclonal, 1:100) and Non-phospho (Active) β-Catenin (#D13A1, rabbit monoclonal, 1:500) were purchased from Cell Signalling Technology. Retrovirus generation and infection Retroviruses expressing shRNA for Tgrbr2 , and Cdkn2 , were constructed using a modified pMSCV vector (Clontech) [56] . For shRNA constructs for Tgfbr2 (Tgfbr2-sh1, -sh2 and -sh3) and Cdkn2a (Cdkn2a-sh1 and -sh2), the following sequences were synthesized and subcloned into pMSCV-EGFP: Cdkn2a-sh1, 5′-GATGATGATGGGCAACGTTCACTCGAGTGAACGTTGCCCATCATCATC-3′; Cdkn2a-sh2, 5′-CTAGCGATGCTAGCGTGTCTACTCGAGTAGACA CGCTAGCATCGCTAG-3′; Tgfbr2-sh1, 5′-TGGCAGAAATTACAAGTGCATATTTCTCGAGAAATATGCACTTGTAATTTCTGCCA-3′; Tgfbr2-sh2, 5′-GTGTAAATACGAATAGCTATGTTCT CGAGAACATAGCTATTCGTATTTACACAC-3′ Tgfbr2-sh3, 5′-GTGGAGGAAGAACGACAAGAACATTCTCGAGAATGTTCTTGTCGTTCTTCCTCCAC-3′. Statistical analysis Values are expressed as means±s.e.m. Statistical significance between two groups was determined by unpaired Student’s t -test. The effect of the TGF-β inhibitor on occurrence of cell death in cKO was determined by χ 2 -test. Data availability ChIP-seq and microarray data that support the findings of this study have been deposited in NCBI GEO with the primary accession codes GSE67132 and GSE66862, respectively. How to cite this article : Mirzamohammadi, F. et al . Polycomb repressive complex 2 regulates skeletal growth by suppressing Wnt and TGF-β signalling. Nat. Commun. 7:12047 doi: 10.1038/ncomms12047 (2016).